Genomic dissection of endemic carbapenem resistance reveals metallo-beta-lactamase dissemination through clonal, plasmid and integron transfer Infections caused by metallo-beta-lactamase-producing organisms (MBLs) are a global health threat. Our understanding of transmission dynamics and how MBLs establish endemicity remains limited. We analysed two decades of bla IMP-4 evolution in a hospital using sequence data from 270 clinical and environmental isolates (including 169 completed genomes) and identified the bla IMP-4 gene across 7 Gram-negative genera, 68 bacterial strains and 7 distinct plasmid types. We showed how an initial multi-species outbreak of conserved IncC plasmids (95 genomes across 37 strains) allowed endemicity to be established through the ability of bla IMP-4 to disseminate in successful strain-genetic setting pairs we termed propagators, in particular Serratia marcescens and Enterobacter hormaechei . From this reservoir, bla IMP-4 persisted through diversification of genetic settings that resulted from transfer of bla IMP-4 plasmids between bacterial hosts and of the integron carrying bla IMP-4 between plasmids. Our findings provide a framework for understanding endemicity and spread of MBLs and may have broader applicability to other carbapenemase-producing organisms. Carbapenemase-producing organisms (CPOs) are now endemic in many regions. While there has been a significant focus on bla KPC due to its spread through North America and Europe, metallo-beta-lactamases (MBLs) (e.g. bla NDM , bla IMP and bla VIM ) are endemic through much of Asia and Oceania including Australia, where bla IMP carbapenemases have dominated [1] , [2] , [3] , [4] , [5] , [6] , [7] , [8] , [9] . Treatment options for infections caused by CPOs, particularly MBL-harbouring organisms, remain severely limited, highlighting the need to stop further spread of these extensively drug-resistant organisms. The mechanisms for carbapenemase spread differ according to carbapenemase type. Some carbapenemases spread through close associations with successful strains or lineages (e.g. bla KPC-2/3 and Klebsiella pneumoniae clonal complex 258), while for others, spread is mediated through association with specific plasmids (e.g. bla OXA-48 and broad-host range IncL plasmids) [10] , [11] . Notably, MBLs spread through both lineage-related clonal expansion and diverse plasmid types [12] , [13] . While surveillance studies have captured some of these data, there have been few efforts to assess how these mechanisms of spread evolve over time. Understanding the transmission dynamics of carbapenem resistance genes will be crucial to inform future infection prevention efforts. Previous work from our group and others have identified that the spread of MBLs, and particularly bla IMP-4 , is often driven by dissemination by transposons of a class 1 integron that has been able to insert into several genetic settings (henceforth defined as either chromosomal integration or different plasmid types carrying bla IMP-4 ) [2] , [4] , [6] , [9] , [14] , [15] . Furthermore, the gene cassettes (such as that carrying bla IMP-4 ) may also be a source of dissemination by being able to enter different class 1 integrons [16] . The ability to study horizontal gene transfer has been significantly advanced by long-read sequencing, which enables high-quality de novo assembly of bacterial genomes, including highly repetitive regions such as plasmids. Utilising long-read sequencing to generate completed, closed bacterial genomes provides a unique opportunity to study the complex, multi-level (bacterial strain, plasmid, gene) transmission dynamics that are likely occurring during MBL spread. When combined with short-read sequencing data, an unprecedented level of detail of the genetic context and likely mechanisms of an outbreak or endemicity is possible. MBL-producing Gram-negative bacteria, dominated by bla IMP-4 , have been isolated in our institution (The Alfred Hospital) since 2002 [5] , [6] , [7] , [15] . After an initial outbreak period in 2004–2005, we experienced hyperendemicity, with a repeated outbreak period from 2017–2020. We aimed to assess the genetic settings of bla IMP-4 , its evolution over time, and the transmission pathways that resulted in repeated outbreaks and endemicity. In this work we used long- and short-read whole genome sequencing to characterise the genetic settings of bla IMP-4 in bacterial chromosomes and plasmids from 277 clinical and environmental isolates from 2002–2020. This allowed us to track the spread of bla IMP-4 in 7 plasmid types and multiple chromosomal settings. In the 18-year period, we noted incredible plasticity of bla IMP-4 persistence, with vertical spread through the transmission of dominant strains and horizontal spread of both plasmids and the class 1 integron carrying bla IMP-4 . We also identified a persistent reservoir of bla IMP-4 in IncC plasmids in both clinical and environmental isolates. Our findings highlight the need for integration of long-read sequencing into CPO surveillance, as well as for multi-modal infection prevention approaches that address the diverse forms of CPO spread. bla IMP-4 found in diverse clinical and environmental isolates spanning two decades We sequenced 277 bla IMP-4 -harbouring isolates from an institutional collection of carbapenem-resistant isolates systematically collected from 2002–2020, including 264 clinical isolates from 196 patients and 13 environmental isolates (Supplementary Dataset 1 ). This included short-read (Illumina) data on all isolates and long-read (Oxford Nanopore) data on 172 isolates that best represented the strains across the study time periods. Seven isolates failed quality control and were excluded. In total, we analysed 270 isolates that were made up of 68 bacterial strains (defined as unique species/multi-locus sequence type [MLST] combinations) from 7 Gram-negative genera, highlighting the diversity of bacterial hosts for bla IMP-4 (Fig. 1a ). The five most frequent strains accounted for 190/270 (70%) genomes and included Serratia marcescens (52/270 isolates, 19%) , Enterobacter hormaechei ST190 (44/270 genomes, 17%), E. hormaechei ST93 (36/270 genomes, 13%), Pseudomonas aeruginosa ST111 (35/270 genomes, 13%) and E. hormaechei ST114 (23/270 genomes, 9%) (Fig. 1a ). In addition to bla IMP-4 , 8/270 (3%) genomes carried other carbapenemase genes (4 bla OXA-58 , 2 bla NDM-7 , 1 bla NDM-1 , 1 bla KPC-2 , 1 bla OXA-500 ) and 121/270 (44%) carried mcr-9.1 , a novel determinant of colistin resistance [14] (Supplementary Dataset 1 ). Fig. 1: Summary of bacterial host species, multi-locus sequence types and genetic settings of bla IMP-4 in sequenced isolates. a Pie chart showing key bacterial host strains of bla IMP-4. bla IMP-4 was noted in 7 bacterial genera and 68 bacterial host strains. b Genetic settings and bacterial host species of bla IMP-4 over course of study, as defined by three distinct periods. Abbreviations: No number, Lin lineage, ST sequence type. Full size image bla IMP-4 detected in multiple plasmid and chromosomal genetic settings across three distinct time periods We first determined the genetic setting of bla IMP-4 using 169 completed, circularised genomes (three non-circularised genomes were excluded). bla IMP-4 -carrying plasmids were clustered using MOB-typer [17] , which uses a whole-sequence-based typing system to provide cluster codes for reconstruction and tracking of plasmids. Representative plasmids from each cluster were then used as references for mapping of the 99 genomes with short-read data only and the three non-circularised genomes (Supplementary Dataset 1 ). Overall, 230 and 40 isolates carried bla IMP-4 on a plasmid or on the chromosome, respectively, with seven distinct plasmid types identified and chromosomal integration in multiple strains (Fig. 1b and Supp. 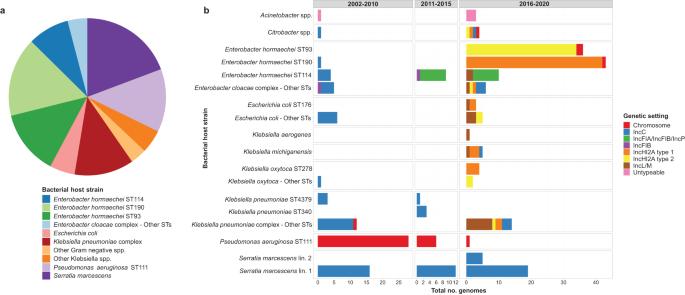Fig. 1: Summary of bacterial host species, multi-locus sequence types and genetic settings ofblaIMP-4in sequenced isolates. aPie chart showing key bacterial host strains ofblaIMP-4.blaIMP-4was noted in 7 bacterial genera and 68 bacterial host strains.bGenetic settings and bacterial host species ofblaIMP-4over course of study, as defined by three distinct periods. Abbreviations: No number, Lin lineage, ST sequence type. Table 1 ). No genomes showed concurrent chromosomal integration and plasmid carriage of bla IMP-4 . For the majority of isolates (151/169, 89%), bla IMP-4 was situated in a class 1 integron most commonly comprising the bla IMP-4 - qacG - aacA4 - catB3 - qacE - sul1 cassette array. The bacterial host strain-plasmid relationships evolved over the course of the study, with three distinct time periods (Fig. 1b ). Outbreak initiation and establishment of bla IMP-4 endemicity bla IMP-4 was first noted in a clinical S. marcescens isolate in 2002, with bla IMP-4 being carried on an IncC plasmid (Supp. Fig. 1 ). It took ~2 years before further bla IMP-4 -carrying Gram-negative bacteria were identified, and these were dominated by an IncC genetic setting or chromosomal bla IMP-4 in P. aeruginosa (Fig. 1b ). Notably, the first S. marcescens lineage (here called lineage 1) with IncC-carrying bla IMP-4 became a successful lineage across the entire study period (Fig. 1b ). S. marcescens lineage 1 included 47 genomes from both clinical and environmental (intensive care unit [ICU] sinks) isolates. Based on their genetic relatedness (median pairwise single nucleotide variant [SNV] distance of 8 [IQR 4–11]), vertical transmission was most likely (Fig. 2a and Supp. 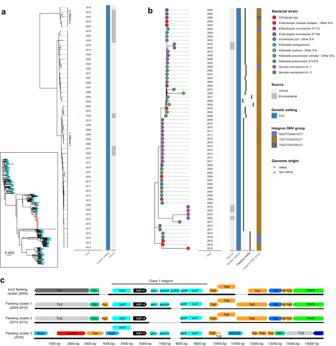Fig. 2: Phylogenetic analysis ofblaIMP-4-carryingS. marcescensand IncC plasmids and analysis ofblaIMP-4flanking regions inPseudomonas aeruginosaST111. aPhylogenetic analysis ofblaIMP-4-carryingS. marcescensgenomes from Alfred Hospital. Inset panel locatesS. marcescensgenomes from the Alfred Hospital in a globalS. marcescensphylogeny. Outer panel shows Alfred Hospital genomes only, indicating that they formed two distinct lineages and were detected both in clinical and environmental samples.bPhylogenetic analysis ofblaIMP-4IncC plasmids using Mashtree. IncC plasmids entered 37 bacterial host strains but remained stable with four flanking region clusters and one integron SNV profile accounting for 93% and 90% plasmids, respectively.cAnalysis ofblaIMP-4flanking regions inP. aeruginosaST111. Three flanking clusters were detected inP. aeruginosaST111. Differences are shown to the class 1 integron present in contemporaneousblaIMP-4IncC plasmids (top), with absence ofcatB3cassette in flanking cluster 1 (in genomes from 2004–2012), absence ofqacG, aac4andcatB3cassettes in flanking cluster 2 (2014–2015) and distinct flanking regions and absence ofcatB3cassette in flanking cluster 3 (2018). Abbreviations: bp base pairs, Lin. lineage, SNV single nucleotide variant, ST sequence type. Table 2 ). The IncC plasmid was rapidly noted in diverse bacterial hosts, with expansion from S. marcescens into 13 other bacterial strains in 2004 alone. Ultimately, this plasmid was noted in 95 genomes across 37 strains (Fig. 2b ), with S. marcescens genomes accounting for the majority (52/95 [54.7%]). Despite the diversity of IncC-carrying bacterial hosts over the 18 years, IncC plasmids were highly conserved, with only 11 SNVs across the plasmid backbone (median pairwise distance of 0 SNVs) (Supp. 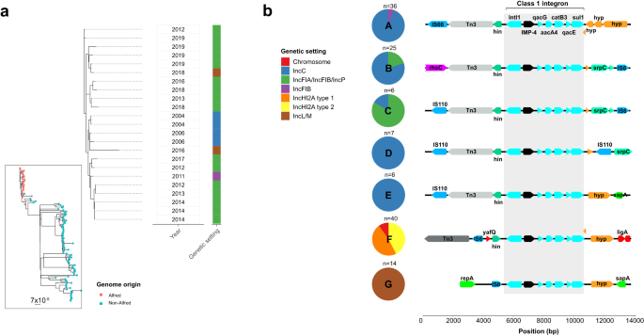Fig. 3: Phylogenetic analysis ofblaIMP-4-carryingE. hormaecheiST114 and clustering analysis ofblaIMP-4-flanking regions. aPhylogenetic analysis ofblaIMP-4-carryingE. hormaecheiST114 genomes from Alfred Hospital. Inset panel placesE. hormaecheiST114 genomes from the Alfred Hospital in a globalE. hormaecheiST114 phylogeny. Outer panel shows Alfred Hospital genomes only. Although clonally related, they were more diverse than other keyblaIMP-4bacterial host strains and were able to act as versatile acceptors ofblaIMP-4in different genetic settings, including four different plasmid types throughout the study.bClustering analysis of flanking regions 5000 bp upstream and downstream ofblaIMP-4using Flanker. The six key flanking region clusters with >5 genomes are shown on the left and the genetic context is shown on the right. IncFIB and IncFIA/IncFIB/IncP plasmids clustered with IncC plasmids throughout the analysis and shared homology both upstream and downstream ofblaIMP-4. Abbreviations: bp. base pairs, SNV single nucleotide variant. Table 3 ) and almost all (70/71, 98.5%) IncC plasmids belonged to the same MOB-typer primary/secondary clusters (AA860 AJ266, Supp. Table 1 ). We noted seven IncC mosaic plasmids with additional replicon types that were excluded from further clustering analyses (Supp. 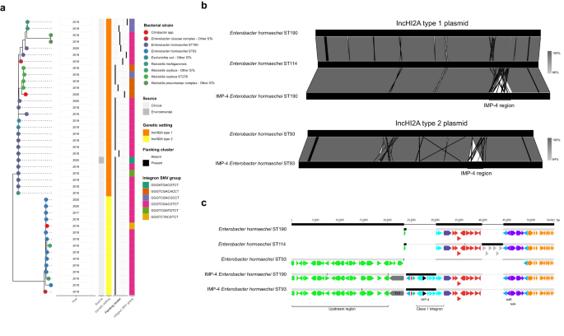Fig. 4: Phylogenetic analysis ofblaIMP-4-carrying IncHI2A plasmids and comparison to non-blaIMP-4IncHI2A plasmids. aPhylogenetic analysis of IncHI2A plasmids using Mashtree. Two distinct plasmid types (IncHI2A type 1 and type 2) were noted from 2016–2020 and rapidly entered 15 bacterial strains. These plasmids shared flanking regions and integron SNV profiles, which were distinct to those noted in other plasmid types.b,cComparative analysis ofblaIMP-4-carrying IncHI2A plasmids to non-blaIMP-4IncHI2A plasmids fromE. hormaecheiST190, ST93 and ST114 from Alfred Hospital. IncHI2A type 1 plasmids fromE. hormaecheiST190 had homology over 100% of the non-blaIMP-4plasmid, with the addition of a 33 kbp region carrying the class 1 integron in theblaIMP-4plasmid. IncHI2A type 2 plasmids fromE. hormaecheiST93 shared homology across 97.6% of the non-blaIMP-4plasmid, with theblaIMP-4integron contained in a mosaic region. Abbreviations: bp base pairs, SNV single nucleotide variant, ST sequence type. Table 4 ). Fig. 2: Phylogenetic analysis of bla IMP-4 -carrying S. marcescens and IncC plasmids and analysis of bla IMP-4 flanking regions in Pseudomonas aeruginosa ST111. a Phylogenetic analysis of bla IMP-4 -carrying S. marcescens genomes from Alfred Hospital. Inset panel locates S. marcescens genomes from the Alfred Hospital in a global S. marcescens phylogeny. Outer panel shows Alfred Hospital genomes only, indicating that they formed two distinct lineages and were detected both in clinical and environmental samples. b Phylogenetic analysis of bla IMP-4 IncC plasmids using Mashtree. IncC plasmids entered 37 bacterial host strains but remained stable with four flanking region clusters and one integron SNV profile accounting for 93% and 90% plasmids, respectively. c Analysis of bla IMP-4 flanking regions in P. aeruginosa ST111. Three flanking clusters were detected in P. aeruginosa ST111. Differences are shown to the class 1 integron present in contemporaneous bla IMP-4 IncC plasmids (top), with absence of catB3 cassette in flanking cluster 1 (in genomes from 2004–2012), absence of qacG, aac4 and catB3 cassettes in flanking cluster 2 (2014–2015) and distinct flanking regions and absence of catB3 cassette in flanking cluster 3 (2018). Abbreviations: bp base pairs, Lin. lineage, SNV single nucleotide variant, ST sequence type. Full size image We used Mashtree [18] to further characterise relatedness of the 64 non-mosaic IncC plasmids, which highlighted the similarity of plasmids across bacterial hosts and different time periods (Fig. 2b ). This was also reflected in the bla IMP-4 flanking regions and integron sequences. Cluster analysis of the flanking regions up to 5000 bp upstream and downstream of bla IMP-4 using Flanker [19] identified only four flanking regions (excluding singletons) in IncC plasmids, accounting for 67/71 (94%) genomes (Fig. 2b ). The bla IMP-4 containing integrons in the IncC plasmids were also highly similar, with a single SNV profile (TGGTCGACGCCT) accounting for 63/69 (91%) plasmids with intact integrons (Fig. 2b ). Taken together, these findings suggest that bla IMP-4 containing IncC plasmids dominated the early outbreak period and established endemicity through their ability to rapidly spread across different bacterial hosts while maintaining stability. S. marcescens was a persistent host and reservoir for bla IMP-4 IncC during this time period (2002–2010) (Supp. Fig. 1 ). In addition to bla IMP-4 IncC plasmids, chromosomal integration of bla IMP-4 into P. aeruginosa ST111 (a global MDR lineage) [20] was also a dominant feature of this early time period (Fig. 1b and Supp. Fig. 1 ). These isolates were rapidly noted in nine patients in 2004 and continued to be isolated until 2018. The pseudomonal isolates were highly related (mean pairwise SNV distance of 1.6 SNVs vs 38.7 SNVs between Alfred and publicly available ST111 genomes [ P < 0.001]) (Supp. Fig. 2a ) but the bla IMP-4 containing integron and the flanking regions differed depending on the time period of isolation, and were also different to the integron and flanking region sequence of the IncC plasmids (Fig. 2c ). Despite being temporally associated, the chromosomal integration of bla IMP-4 in P. aeruginosa ST111 with a different integron structure and flanking regions suggests that bla IMP-4 entry into P. aeruginosa likely arose independently of the bla IMP-4 IncC plasmids. Low endemicity of bla IMP-4 and entry into novel plasmids Apart from ongoing isolation of bla IMP-4 IncC plasmids (predominately in S. marcescens ) and chromosomal bla IMP-4 P. aeruginosa , the evolution of the following time period (2011–2015) was characterised by bla IMP-4 entering novel plasmids in E. hormaechei ST114 (a global MDR nosocomial Enterobacter clone) [21] (Fig. 1b and Supp. Fig. 1 ). At the start of the outbreak, there were a small number of E. hormaechei ST114 with bla IMP-4 -carrying IncC plasmids, but during this period, E. hormaechei ST114 acquired bla IMP-4 -carrying IncFIB and IncFIA/IncFIB/IncP plasmids (Fig. 1b ). Phylogenomic analysis showed that the E. hormaechei ST114 isolates were more diverse (median pairwise SNV distance 35, IQR 27–46) but the Alfred Hospital isolates still clustered more closely than other publicly available genomes (Fig. 3a and Supp. Table 2 ). To determine if the IncC plasmids were the source of bla IMP-4 in the IncFIB and IncFIA/IncFIB/IncP plasmids, we analysed the bla IMP-4 flanking regions across the three plasmids (Fig. 3b ). We noted homology of the 3850 bp upstream and 305 bp downstream regions of the integron in IncC, IncFIA/IncFIB/IncP and IncFIB plasmids (clusters A, B and C) with Tn3 transposons and DNA recombinases ( hin) located immediately upstream. (Fig. 3b ). These three plasmids also shared the same integron SNV profile (TGGTCGACGCCT) (Supp. Fig. 3 ). Taken together, these findings suggested that as the bla IMP-4 -harbouring IncC plasmids became endemic during the first time period (2002–2010), the outbreak evolved whereby the IncC plasmids served as a bla IMP-4 reservoir not only for inter-strain plasmid transfer, but also transfer of the bla IMP-4 integron and flanking regions between IncC, IncFIA/IncFIB/IncP and IncFIB plasmids. Fig. 3: Phylogenetic analysis of bla IMP-4 -carrying E. hormaechei ST114 and clustering analysis of bla IMP-4 -flanking regions. a Phylogenetic analysis of bla IMP-4 -carrying E. hormaechei ST114 genomes from Alfred Hospital. Inset panel places E. hormaechei ST114 genomes from the Alfred Hospital in a global E. hormaechei ST114 phylogeny. Outer panel shows Alfred Hospital genomes only. Although clonally related, they were more diverse than other key bla IMP-4 bacterial host strains and were able to act as versatile acceptors of bla IMP-4 in different genetic settings, including four different plasmid types throughout the study. b Clustering analysis of flanking regions 5000 bp upstream and downstream of bla IMP-4 using Flanker. The six key flanking region clusters with >5 genomes are shown on the left and the genetic context is shown on the right. IncFIB and IncFIA/IncFIB/IncP plasmids clustered with IncC plasmids throughout the analysis and shared homology both upstream and downstream of bla IMP-4 . Abbreviations: bp. base pairs, SNV single nucleotide variant. Full size image Hyperendemicity and repeat outbreaks driven by clonal expansion of new bacterial strains and inter-species plasmid spread The most recent time period (2016–2020) was characterised by complex, multi-level transmission dynamics resulting from the emergence of several new and highly successful bla IMP-4 plasmids and clonal expansion of E. hormaechei ST190 and ST93 host strains (Fig. 1b ). Ongoing circulation of bla IMP-4 in genetic settings and bacterial strains from prior periods was also observed (Fig. 1b ). Early in this period, bla IMP-4 was identified in a new plasmid, IncL/M, first in E. hormaechei ST114, which was its fourth bla IMP-4 carrying plasmid, and then in a wide range of other bacterial strains ( n = 16) (Fig. 1b ). All IncL/M plasmids belonged to the same MOB-typer cluster, shared the same SNV profile in the integron (GGGTCGACGCCT) and 14/17 shared the same flanking cluster (Cluster G) (Fig. 3b ). The three plasmids with other flanking clusters had minor variations in the Cluster G flanking region leading to them being clustered as singletons. These flanking regions were distinct from all other bla IMP-4 plasmids, however the same integron SNV profile was also noted in other plasmids (Supp. 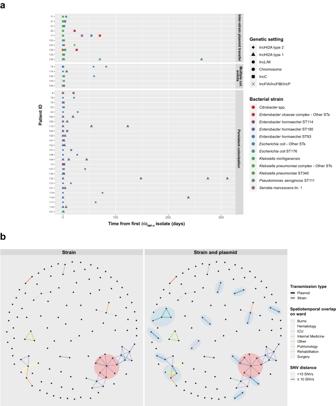Fig. 5: Within-patient longitudinal analysis ofblaIMP-4spread and between-patientblaIMP-4transmission analysis. aLongitudinal analysis ofblaIMP-4in patients with multiple genomes available. Each line represents a patient with colours representing the bacterial host and shapes representing theblaIMP-4genetic setting.bAnalysis of potential transmission events between patients. Individual patients are shown as vertices. Edges were drawn if there was spatiotemporal overlap on a hospital wards (indicated by edge colour) and a genomic criterion was met. In the left panel, the genomic criterion was having the sameblaIMP-4bacterial strain with SNV distance from phylogenetic analysis indicated by shading. In the right panel, the genomic criterion incorporated both the strain transmission analysis as well as detecting presence ofblaIMP-4in the same plasmid (as defined by MOB-typer cluster) in different bacterial strains. The additional benefit of plasmid analysis is indicated by the blue shading of the potential transmission events in this panel. The red shading indicates the patient with the highest betweenness-centrality and their contacts. Abbreviations: ICU intensive care unit, Lin. lineage, SNV single nucleotide variant, ST sequence type. Table 5 and Supp. Fig. 3 ). In 2017, bla IMP-4 was detected for the first time in IncHI2A plasmids in a small outbreak of Klebsiella oxytoca ST278 and Klebsiella michiganensis ST50 (Fig. 1b ). The first IncHI2A plasmid (type 1—as defined by MOB-typer cluster AA739 AJ055) then spread to E. hormaechei ST190 and a second IncHI2A plasmid (type 2—MOB-typer cluster AA739 AJ058) emerged in E. hormaechei ST93, with both bacterial strains undergoing significant clonal expansion and contributing to a repeated outbreak and hyperendemicity from 2017–2020 (Figs. 1 b and 4a ). Bacterial isolates carrying bla IMP-4 on these two IncHI2A plasmids ultimately accounted for 98/161 (61%) of the sequenced genomes in that period (with 36/98 E. hormaechei ST93 and 43/98 E. hormaechei ST190) (Fig. 4a ). The E. hormaechei ST93 and ST190 bacterial hosts were highly clonal with a median pairwise SNV distance of 9 (IQR 2-14) and 3 (IQR 2–4), respectively (Supp. Fig. 2 b and 2c , Supp. Table 2 ). In addition to these two strains, the IncHI2A plasmids were found in 13 other strains (Fig. 4a ). Analysis of the bla IMP-4 flanking regions and integrons in the IncHI2A plasmids showed the same flanking sequence (Cluster F) across 36/47 (77%) plasmids and the same integron SNV profile (GGGTCGACGTCT) in 35/47 (74%) plasmids across both IncHI2A plasmid types (Fig. 4a ). These flanking sequences and integron SNV profiles were not found in other plasmid types (Supp. Fig. 3 ), suggesting that they may have arisen independently of other bla IMP-4 genetic settings. Fig. 4: Phylogenetic analysis of bla IMP-4 -carrying IncHI2A plasmids and comparison to non- bla IMP-4 IncHI2A plasmids. a Phylogenetic analysis of IncHI2A plasmids using Mashtree. Two distinct plasmid types (IncHI2A type 1 and type 2) were noted from 2016–2020 and rapidly entered 15 bacterial strains. These plasmids shared flanking regions and integron SNV profiles, which were distinct to those noted in other plasmid types. b , c Comparative analysis of bla IMP-4 -carrying IncHI2A plasmids to non- bla IMP-4 IncHI2A plasmids from E. hormaechei ST190, ST93 and ST114 from Alfred Hospital. IncHI2A type 1 plasmids from E. hormaechei ST190 had homology over 100% of the non- bla IMP-4 plasmid, with the addition of a 33 kbp region carrying the class 1 integron in the bla IMP-4 plasmid. IncHI2A type 2 plasmids from E. hormaechei ST93 shared homology across 97.6% of the non- bla IMP-4 plasmid, with the bla IMP-4 integron contained in a mosaic region. Abbreviations: bp base pairs, SNV single nucleotide variant, ST sequence type. Full size image To understand the rapid appearance of bla IMP-4 IncHI2A plasmids, we compared them to carbapenem-susceptible, non- bla IMP-4 IncHI2A plasmids in single E. hormaechei ST114, ST190 and ST93 genomes from our institution. The plasmids were highly similar between bla IMP-4 and non- bla IMP-4 bacterial strains (Fig. 4b ). The IncHI2A type 1 plasmids from bla IMP-4 E. hormaechei ST190 had the addition of a 33 kbp region carrying the class 1 integron with bla IMP-4 (Fig. 4b ). The IncHI2A type 2 plasmids from bla IMP-4 E. hormaechei ST93 shared 97.6% homology with the non- bla IMP-4 plasmid, with the bla IMP-4 integron contained in a mosaic region (Fig. 4b, c ). These data suggested integration of bla IMP-4 into pre-existing carbapenem-susceptible Enterobacter carrying IncHI2A plasmids, with mobilisation of the regions upstream and downstream. These flanking regions in IncHI2A plasmids were distinct to those in other bla IMP-4 plasmids, with a different IS110-like insertion sequence/Tn3 transposon combination (Fig. 4c ). While the arrival of new IncHI2A and IncL/M plasmids was the major contributor to the repeated outbreak and hyperendemicity during this period, we saw ongoing circulation of bla IMP-4 in prior genetic settings. In particular, we saw IncC plasmids circulating (32/161 genomes, 19.9%), including in a novel lineage of S. marcescens in 2019 (lineage 2—Fig. 2a ). We also noted bla IMP-4 -harbouring P. aeruginosa ST111 (1 genome) and E. hormaechei ST114 with bla IMP-4 IncFIA/IncFIB/IncP plasmids (9 genomes). This reflected a cumulative trend where the prior bla IMP-4 genetic settings persisted in the context of new bacterial strains and plasmids, rather than waxing and waning over time. An environmental reservoir of bla IMP-4 plasmids In response to the outbreak in the most recent time period, we conducted environmental screening of ICU sinks from 2019–2020 and cultured 34 bla IMP-4 isolates (33 S. marcescens and one E. hormaechei ), with 11 isolates selected for sequencing. Despite E. hormaechei predominating in bla IMP-4 clinical isolates, 6 genomes were S. marcescens lineage 1, 4 S. marcescens lineage 2, and one E. hormaechei ST190. These genomes closely matched clinical isolates, with bla IMP-4 being located on IncC plasmids and IncHI2A type 1 plasmids in S. marcescens and E. hormaechei ST190, respectively (Figs. 2 b and 4a ). This indicated that sinks were a possible reservoir for bla IMP-4 and may have explained the persistence of S. marcescens with closely matching IncC plasmids throughout the study (Fig. 2b ). Within-patient and between-patient bla IMP-4 analyses show importance of diversification of genetic settings through plasmid transfer Patients with serial bla IMP-4 -harbouring genomes available followed different trajectories of bla IMP-4 carriage (Fig. 5a ). Multiple colonisation events were noted in 5/41 patients, with bla IMP-4 being located in distinct genetic settings (i.e. differing plasmids and/or chromosomal integration). Flanking region/integron SNV profiles also differed, making within-patient integron transfer unlikely. Possible within-patient inter-strain transfer of key bla IMP-4 plasmids (IncC, IncL/M, IncHI2A types 1 and 2) occurred in 10/41 patients with the same bla IMP-4 plasmid types being noted in multiple strains (Fig. 5a ). In 7 patients, the evidence was particularly compelling as plasmids had identical flanking sequences and integron SNV profiles across different bacterial hosts. Persisting colonisation was noted in 26 patients, with the same strain and same bla IMP-4 genetic setting repeatedly isolated. Fig. 5: Within-patient longitudinal analysis of bla IMP-4 spread and between-patient bla IMP-4 transmission analysis. a Longitudinal analysis of bla IMP-4 in patients with multiple genomes available. Each line represents a patient with colours representing the bacterial host and shapes representing the bla IMP-4 genetic setting. b Analysis of potential transmission events between patients. Individual patients are shown as vertices. Edges were drawn if there was spatiotemporal overlap on a hospital wards (indicated by edge colour) and a genomic criterion was met. In the left panel, the genomic criterion was having the same bla IMP-4 bacterial strain with SNV distance from phylogenetic analysis indicated by shading. In the right panel, the genomic criterion incorporated both the strain transmission analysis as well as detecting presence of bla IMP-4 in the same plasmid (as defined by MOB-typer cluster) in different bacterial strains. The additional benefit of plasmid analysis is indicated by the blue shading of the potential transmission events in this panel. The red shading indicates the patient with the highest betweenness-centrality and their contacts. Abbreviations: ICU intensive care unit, Lin. lineage, SNV single nucleotide variant, ST sequence type. Full size image We then used patient movement data (available in 127 patients from 2013 onwards) to establish putative transmission events (Fig. 5b ), defined as spatiotemporal overlap between patients and genomic evidence of potential transmission. For genomic evidence, we considered both strain transmission (same bacterial host strain carrying bla IMP-4 in the same genetic setting) and plasmid transmission (detection of the same plasmid by MOB-typer cluster in different bacterial strains). We linked 71/127 (56%) patients using these definitions and identified the ICU as a major transmission site with 36/76 (47%) potential transmission events across 7/16 (44%) transmission networks, including the two largest networks (23 and 9 patients, respectively). While strain transmission contributed significantly, use of long-read sequencing to detect potential plasmid transmission allowed us to detect an additional 5/10 (50%) wards, 7/16 (44%) transmission networks and link 22/71 (31%) patients beyond what was identified for strain transmission alone (Fig. 5b ). We measured betweenness centrality to identify key patients involved in transmission [22] . The patient with the highest betweenness centrality (164.0 vs mean 4.9) had a > 4-month ICU admission and was implicated in 7 transmission events, placing them at the centre of the large 23-patient network spanning those two strains and plasmid types ( E. hormaechei ST190 with IncHI2A type 1 plasmid and E. hormaechei ST93 with IncHI2A type 2 plasmid) (Fig. 5b ). A further transmission event to a single patient then occurred during an admission on the Cardiology ward 6 months later. The spread of carbapenemases is the major driver of carbapenem resistance globally [23] and has been the focus of numerous cross-sectional studies [12] , [13] , [24] . To date, there have been limited efforts to study carbapenem resistance over extended time periods [25] , [26] . In this study we had a unique opportunity to analyse two decades of bla IMP-4 carbapenemases in our institution and gained important insights into how bla IMP-4 caused outbreaks and perpetuated endemicity. bla IMP-4 spread occurred through multiple mechanisms including strain transmission, plasmid transmission and transfer of the bla IMP-4 class 1 integron. Each of these had a different qualitative and quantitative contribution to bla IMP-4 persisting at our institution, highlighting that endemicity is a nuanced process requiring these mechanisms to act in concert. These findings carry important implications for prevention of future carbapenemase endemicity. From a pathogen perspective, we propose that there are two key conditions required for bla IMP-4 endemicity. Firstly, there is a need for diversification of genetic settings for the resistance determinant, which in our study occurred through extensive inter-strain transmission of key bla IMP-4 plasmids (IncC, IncHIA2 type 1 and type 2, IncL/M), as well as mobilisation by transposons of the class I integron and entry into new plasmids (IncFIB, IncFIA/IncFIB/IncP). This ability to diversify led to the initial establishment of endemicity with IncC plasmids, and also to the period of hyperendemicity due to the emergence of a novel context in IncHI2A and IncL/M plasmids. To study this emergence, we demonstrated that bla IMP-4 IncHI2A plasmids were highly similar to non- bla IMP-4 IncHI2A plasmids in E. hormaechei ST93, ST114 and ST190 that may have served as acceptors for the bla IMP-4 integron. In addition, there was possible importation from outside sources: bla IMP-4 has been found in both IncHI2A and IncL/M plasmids in Australian isolates [2] , [4] , [9] , [27] and bla IMP-4 -harbouring IncHI2A plasmids are emerging as a global issue, having been noted in a recent multi-hospital outbreak in the United Kingdom [28] . The second condition is propagation of bla IMP-4 through the establishment of high-risk strain-genetic setting pairs we term propagators. While we noted bla IMP-4 in 68 strains during the study, five strains accounted for 190/270 (70%) genomes and 140/196 (71%) patients colonised with bla IMP-4 . The first of these was S. marcescens lineage 1 (IncC plasmids), which defined the early period of the study and continued to persist throughout. This propagator pair was able to act as a reservoir of bla IMP-4 , likely through occupying an environmental niche as we noted during sampling of ICU sinks. The colonisation of hospital plumbing by CPOs has been well documented [9] , [29] , [30] , [31] , [32] , including bla IMP-4 -harbouring S. marcescens in an Australian setting that was unable to be eradicated [33] . This environmental colonisation probably enabled clonal spread of bla IMP-4 -harbouring S. marcescens and may have driven diversification through inter-strain transfer of bla IMP-4 IncC plasmids and inter-plasmid transfer of the bla IMP-4 class I integron. Other propagators emerged at various junctures including P. aeruginosa ST111 (chromosome) and E. hormaechei ST114 (IncFIA/IncFIB/IncP plasmids), then E. hormaechei ST190 and ST93 (IncHI2A type 1 and type 2 plasmids, respectively). Clonal spread of propagators was therefore central to establishing and maintaining bla IMP-4 endemicity, as well as leading to a repeated outbreak and hyperendemicity in the final period of the study. These findings broadly fit the ‘multiple lineages, multiple plasmids’ designation proposed by David et al. when analysing carbapenemase spread in K. pneumoniae [12] but we demonstrated that the dynamics of carbapenemase endemicity in our setting were significantly more complex with clonal transmission of propagator strains, inter-strain plasmid transmission and inter-plasmid integron transmission all playing important roles. In addition to pathogen factors, we were able to analyse patient factors. While genomic surveillance previously focused on lineage-level analysis, long-read sequencing technologies have improved analysis of plasmids and other mobile genetic elements [12] , [28] , [34] . In our study, these insights proved informative both for understanding within-patient and between-patient bla IMP-4 spread. Within patients, we detected different trajectories of colonisation. Patients who undergo multiple colonisation events may be at the core of multiple transmission networks, as demonstrated by the patient colonised with two IncHI2A plasmids and highest betweenness centrality. Patients with inter-strain plasmid transfer may facilitate the diversification of genetic settings for bla IMP-4 , thus increasing the risk of newly successful propagators emerging [13] , in turn fuelling outbreaks. Of note, we did not find clear evidence of bla IMP-4 integron transfer events within-patients, suggesting that they may play a lesser role. Long-read technologies also allowed us to analyse putative plasmid transmission between-patients, which implicated an additional 50% of wards, 44% transmission networks and 31% patients over strain transmission alone. We used detection of bla IMP-4 plasmids of the same MOB-typer primary/secondary clusters as a simple definition [17] but quantitative thresholds incorporating changes in plasmid backbones and large-scale recombination events across a diverse array of bacterial hosts, plasmids and resistance determinants are needed [35] . Our study had several limitations. Firstly, it was based on an isolate collection that spanned two decades with some patient data from the early part of the study being incomplete. Similarly, approaches to isolate sampling changed during that time, in particular since the inception of a statewide CPO detection programme that mandated screening in high-risk areas [36] and likely led to increased detection of CPO colonisation in the last 4 years of the study. Finally, our study focused on bla IMP-4 and was from a single centre, which may limit the generalisability of findings to outbreaks at other centres. In summary, we showed that bla IMP-4 endemicity and repeated outbreaks were due to diversification of genetic settings through inter-strain bla IMP-4 plasmid transfer and inter-plasmid bla IMP-4 integron transfer in combination with clonal expansion that led to an evolving cascade of high-risk strain-genetic setting pairs. Our findings provide a framework for understanding endemicity of MBL-producing organisms and may have broader applicability to other CPOs. Our study highlights that stopping the spread of CPOs will require adequate surveillance to detect not only the presence of resistance determinants and their bacterial host strains but also their genetic context and plasmid-integron transmission dynamics, thus enabling early detection of novel and potentially hidden threats. The study was approved by the Alfred Hospital Ethics Committee (Project No: 44/20) with a waiver of consent for patient data due to its retrospective and observational nature. Isolate selection We systematically reviewed an institutional collection spanning all CPO isolates from 2002 to 2020. The collection contained isolates collected as part of routine clinical care, as well as environmental screening of sinks from 2018–2020. Routine antimicrobial susceptibility testing was performed using Vitek2 (BioMérieux). We identified bla IMP-4 carriage through polymerase chain reaction (PCR) screening. GoTaq Flexi DNA polymerase (Promega, Wisconsin, USA) was used as per manufacturer’s instructions and 10 µmol of the primers Imp4_screen_F (5′-CCAGGACACACTCCAGATAACC-3′) and Imp4_screen_R (5′-CAAGAGTGATGCGTCTCCAGC-3′) in 25 μL reaction volumes. PCR was performed using the following cycle conditions: 98 °C for 2 min, followed by 30 cycles of 98 °C for 30 sec, 55 °C for 30 sec, 72 °C for 30 sec. Amplicons were resolved by agarose gel electrophoresis on a 1% w/v agarose gel. We selected 277 bla IMP-4 isolates for whole genome sequencing (WGS) based on bacterial strain (species/MLST combination) and year of isolation. For species with <30 isolates, we sequenced all available isolates. For species with >30 isolates, we performed WGS on selected isolates based on collection date to ensure that we had sequencing data available for all study periods. We sequenced at least one isolate of all strains across all study periods with both short-read (Illumina) and long-read (Oxford Nanopore) technologies ( n = 172). We also selected one carbapenem-susceptible E. hormaechei ST93 and one E. hormaechei ST190 isolate for short- and long-read WGS. Culture, DNA extraction and sequencing All bacterial isolates were grown on cation-adjusted Mueller-Hinton II agar (Becton-Dickinson) for 16 h at 37 °C, and sub-cultured into cation-adjusted Mueller-Hinton broth (Becton-Dickinson) for a further 16 h at 37 °C. Bacterial genomic DNA was extracted from liquid culture using the GenFind V3 Reagent Kit (Beckman Coulter) as per manufacturer’s instructions. Libraries for short read sequencing were prepared using the Nextera Flex DNA Library Prep Kit (Illumina), and 150 bp paired-end sequencing was performed on the NovaSeq 6000 system (Illumina). Libraries for long-read sequencing were prepared using the Ligation Sequencing Kit with Native Barcoding Expansion (Oxford Nanopore Technologies) and sequenced on the MinION instrument with an R9.4.1 flow cell (Oxford Nanopore Technologies) for 48 h. Basecalling was performed with Guppy v.4.0.14 using the ‘high accuracy’ basecalling model. De novo assembly and annotation We constructed de novo assemblies of all isolates with only short-read data using the Shovill v1.0.4 wrapper for SPAdes, which also utilizes Trimmomatic for read trimming and Pilon for read error correction [37] , [38] , [39] , [40] . For long-read assembly, long reads were filtered using Filtlong v.0.2.0 [41] with the following parameters: ‘--min_length 1000 --keep_percent 90 --target_bases 500000000’. Hybrid assemblies incorporating short- and long-read data were created using Unicycler v.0.4.08 with standard parameters [42] with Unicycler output used to assess circularisation. If bla IMP-4 contigs were non-circularised, we re-assembled genomes using a long-read-first assembly using a bespoke pipeline ( https://github.com/HughCottingham/clinopore-nf ) that incorporates Flye v2.9.2 with subsequent polishing with Medaka v1.8.0, Polypolish v0.5.0 and Polca v3.4.1 [43] , [44] , [45] , [46] . Assembly quality was checked using Quast [47] v5.2.0 and species identification was performed using GTDB-Tk [48] v1.0.2 and checked against isolate identification performed at time of isolate collection. We excluded genomes ( n = 7) with a species mismatch, as well as genomes whose assemblies had >1000 contigs, N50 < 10,000 or assembly length >7.5 Mb. On the remaining assemblies ( n = 270), we annotated the genomes using Prokka v1.14.6 [49] . We then performed resistance gene and plasmid replicon detection with Abricate v.1.0.0 [50] , using the NCBI Antibiotic Resistance and PlasmidFinder databases, respectively. We determined in silico multi-locus sequence type (ST) using ‘mlst’ v.2.19.0 [51] . All inconclusive ST calls with ‘mlst’ were checked with SRST2 [52] v0.2.0. Core genome-based phylogenetic analyses We performed core genome-based phylogenetic analyses on key STs, defined as those with ≥5 isolates available from our institution. This included E. hormaechei ST93, ST114, and ST190 and P. aeruginosa ST111. Due to the absence of an MLST schema for S. marcescens we identified all RefSeq S. marcescens genomes and used Assembly Dereplicator v0.1.0 ( https://github.com/rrwick/Assembly-Dereplicator ) with a Mash distance threshold of 0.001 to remove duplicate assemblies. We then used these assemblies, in conjunction with S. marcescens genomes from our institution to construct a phylogeny using Mashtree [18] v1.2.0. In brief, this tool uses non-alignment based assessment of sequence similarity through use of the min-hash algorithm, as implemented in Mash [53] , to generate distance metrics between input sequences. These are then used to cluster sequences using the neighbour joining algorithm. This allowed us to identify that Alfred Hospital genomes belonged to two lineages, for which we conducted the same phylogenetic analyses as we did within STs for other species. This consisted of identifying RefSeq genomes of the same ST and including them for context in phylogenetic analyses. We chose one completed, closed assembly from our institution for each ST to use as a reference. Mobile genetic elements were excluded from these reference assemblies using PHASTER and IslandViewer 4 [54] , [55] . A core chromosomal SNV alignment was generated using Snippy v.4.6.0 [56] and recombination was removed using Gubbins [57] v3.3. We then used this core genome alignment in IQtree v.2.0.3 to generate maximum likelihood phylogenies for each ST [58] , with the best-fit model chosen using ModelFinder [59] . For each ST, median SNV distances between isolates from our institution were then calculated. Phylogenetic trees were visualized and annotated with metadata using ‘ggtree’ [60] with additional editing in Adobe Illustrator v2020.24.3. Plasmid phylogenetic analyses Using Abricate, we identified bla IMP-4 -harbouring contigs that were putative plasmids in our hybrid assemblies. We then used the MOB-typer v1.4.9 tool to determine plasmid replicons present, as well as to assign clusters [17] . In addition, we used COPLA [61] to assign plasmid taxonomic units to key plasmid types as determined by MOB-typer. We identified possible mosaic plasmids resulting from fusion events by examining plasmid replicon content within MOB-typer cluster and identifying plasmids which had presence of additional plasmid replicons then manually inspecting the assemblies. We then conducted analyses within key plasmid groups within our dataset, as determined by MOB-typer cluster. These included IncC, IncHI2A type 1, IncHI2A type 2, IncFIA/IncFIB/IncP, IncFIB, IncL/M, and untypeable plasmids from Acinetobacter spp. In order to identify SNVs in the plasmid backbone, we used Snippy v.4.6.0 [56] to create a core SNV alignment by mapping short reads to a reference plasmid from our institution from each plasmid group. We then used Mashtree [18] to generate distance metrics between plasmids belonging to the same group, excluding mosaic plasmids. The R package ‘ggtree’ v3.0.4 was used to visualize the resulting trees [60] and to annotate with metadata. Adobe Illustrator v2020.24.3 was used to merge different parts of the figures together. We also used fastANI v1.3 to generate pairwise average nucleotide identities between plasmids belonging to the same plasmid group [62] . We used progressiveMauve v2.4.0.r4736 to align all plasmids within a plasmid group and assess for structural re-arrangements [63] , then visualized this in Easyfig v2.2.2 [64] . Analysis of bla IMP-4 integron and flanking sequences We used Flanker [19] v0.1.5 to identify and cluster flanking sequences around bla IMP-4 from hybrid contigs. We performed clustering 5000 bp upstream and downstream of the bla IMP-4 gene across windows in 500 bp increments. Geneious v10.2.6 ( https://www.geneious.com ) was used to visualize and assess for structural re-arrangements, with subsequent manual annotation in Adobe Illustrator v2020.24.3. We also assessed for SNVs in the bla IMP-4 integron by aligning bla IMP-4 genetic settings from completed, circularised assemblies to a previously reported bla IMP-4 integron (GenBank accession number JX101693) [4] using MUSCLE v3.8.1551 [65] . Assemblies with large scale insertions or deletions in the integron were excluded (e.g. P. aeruginosa ST111 genomes). We extracted SNVs from the resulting alignment using SNP-sites v2.5.1 [66] and grouped plasmids according to the SNV profile. Short-read mapping to plasmid sequences For genomes which only had short-read data available, we created a database of plasmids from all MOB-typer clusters (described above) and used the Nextflow implementation of the REDDog pipeline (V1.beta10.3; available at https://github.com/scwatts/reddog-nf ) to map short-reads to this database. We used the following parameters: ‘mapping_cover_min = 1, mapping_mapped_min = 0.5, mapping_depth_min = 10’ then analysed the data. A read set was considered to have a match to a plasmid in the database if there was >90% coverage of the plasmid with <10 SNVs. Patient data and transmission events Clinical data were extracted from the electronic medical record. Clinical data were missing for 7 isolates from 2009–2012. Patient movement data were available from 2013 onwards, including 127/196 (65%) patients in the study. As patients did not undergo systematic surveillance for bla IMP-4 , we considered that the patient may have been colonised in the 30 days prior to the first isolation of a bla IMP-4 -harbouring organism and identified overlaps on the same ward at the same time as potential transmission events between patients. We then applied genomic criteria to further confirm potential transmission events. In the first instance, patients would have to have bla IMP-4 -harbouring bacteria of the same strain for a potential transmission event to be considered. These events were then further classified on basis of SNV distance, with a cutoff of 10 SNVs. In the second instance, patients would have to have bla IMP-4 in the same genetic setting (defined as the same MOB-typer primary/secondary cluster), as determined either through completed assemblies or by having a match to a reference plasmid using the short-read mapping approach described above. We then used the R package ‘ggraph’ v2.0.5 to visualize putative transmission networks with patients as nodes and potential transmission events as edges. Betweenness centrality was calculated using the ‘betweenness’ function in the ‘iGraph’ R package (v1.2.11) [67] . Statistical analysis Categorical variables were compared using χ2 or Fisher’s exact tests and continuous variables were compared using Student’s t- test or Mann–Whitney–Wilcoxon, as appropriate. Statistical analyses were performed in R (v4.1.1). Reporting summary Further information on research design is available in the Nature Portfolio Reporting Summary linked to this article.